Siva1 inhibits p53 function by acting as an ARF E3 ubiquitin ligase The tumour suppressor alternative reading frame (ARF) is one of the most frequently mutated proteins in human cancer. It has been well established that ARF is able to stabilize and activate p53 by directly inhibiting Mdm2. ARF-mediated p53 activation in response to oncogenic stress is thought to be an important determinant of protection against cancer. However, little is known regarding the control of ARF in cells. Here, we show that Siva1 is a specific E3 ubiquitin ligase of ARF. Siva1 physically interacts with ARF both in vitro and in vivo. Through direct interaction, Siva1 promotes the ubiquitination and degradation of ARF, which in turn affects the stability of p53. Functionally, Siva1 regulates cell cycle progression and cell proliferation in an ARF/p53-dependent manner. Our results uncover a novel regulatory mechanism for the control of ARF stability, thereby revealing an important function of Siva1 in the regulation of the ARF-Mdm2-p53 pathway. Alternative reading frame (ARF) and p53 are among the most important tumour suppressors based on their frequent and ubiquitous inactivation in human cancer. The tumour suppressor ARF ( p14 ARF in human and p19 ARF in mouse), which is one of the products of the Ink4a/Arf locus (also known as Cdkn2a locus) [1] , acts as a major positive regulator of p53 by binding to Mdm2, the major E3 ligase that is responsible for p53 ubiquitination and degradation [2] , [3] , [4] , [5] , [6] . ARF participates in various p53-related cellular responses [7] , [8] , such as cell cycle arrest, senescence and apoptosis. The ARF/p53 pathway protects cells from several types of damage [9] , [10] , forming the basis of its tumour suppressor activity. ARF protein is generally stable in the nucleolus but rapidly turns over in the nucleoplasm [11] . Although human p14ARF protein is lysine free, it can still be polyubiquitinated and degraded via the proteasome system [12] . Recently, a new E3 ubiquitin ligase (TRIP12/ULF) of ARF has been identified and appears to promote the lysine-independent ubiquitination and degradation of ARF [13] . Siva1, which was initially identified as a protein associated with the cytoplasmic tail of CD27 ( [14] ), is able to bind to Bcl-XL and antagonize UV-induced apoptosis [15] . Further analysis has revealed that Siva1 is a direct transcriptional target of p53 ( [16] ) and is involved in p53-mediated apoptosis [17] . Our recent work has shown that Siva1 acts as a suppressor of p53 activity by facilitating Mdm2-mediated p53 degradation [18] , [19] . In this study, we report that Siva1 is a novel E3 ubiquitin ligase of ARF, and that Siva1 directly regulates the stability of ARF. Via direct interaction, Siva1 promotes the ubiquitination and degradation of ARF. Deletion analysis of Siva1 and ARF suggests that the C terminus of Siva1 and the N terminus of ARF are required for their interaction. Moreover, knockdown of Siva1 stabilizes ARF and p53, while the ectopic expression of Siva1 destabilizes ARF and p53. Furthermore, Siva1 regulates cell cycle progression and cell proliferation in an ARF/p53-dependent manner. Collectively, these results reveal a novel function of Siva1 in the regulation of the ARF-p53 pathway. Siva1 interacts with ARF Our recent work has shown that Siva1 has an important function in the negative regulation of p53 ( [18] ). To further investigate the detailed mechanism, we examined the association between Siva1 and several p53 regulators. Intriguingly, ARF was revealed to be a novel Siva1-binding partner. Co-immunoprecipitation analysis showed that green fluorescent protein (GFP)-ARF specifically binds to Flag-Siva1 ( Fig. 1a ). In contrast, GFP-Siva1 but not the control GFP interacted with Flag-ARF ( Fig. 1b ). The binding of ARF and Siva1 appeared to be direct, as shown by a GST-pull down assay using purified recombinant proteins ( Fig. 1c ). 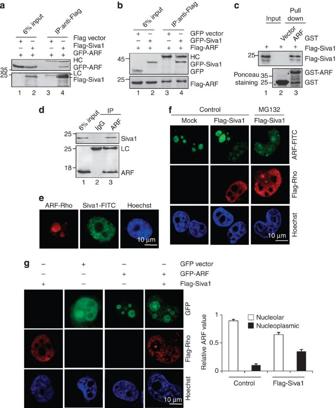Figure 1: Siva1 is a novel ARF-binding partner. (a) H1299 cells were co-transfected with Flag-Siva1 and GFP-ARF as indicated. Twenty-four hours after transfection, cells were treated with 25 μM MG132 for an additional 8 h. The cell lysates were immunoprecipitated with anti-Flag antibody followed by western blot analysis with the indicated antibodies. HC and LC indicate the IgG heavy chain and the IgG light chain, respectively. (b) H1299 cells were co-transfected with GFP-Siva1 and Flag-ARF. Twenty-four hours post transfection, the cells were treated with 25 μM MG132 for an additional 8 h. The cell lysates were subject to immunoprecipitation with anti-Flag antibody. The immunoprecipitates were analysed via western blot analysis. HC indicates the IgG heavy chain. (c) The purified GST and GST-ARF proteins were incubated separately with recombinant Flag-Siva1 protein purified from HEK293T cells. Bead-bound and input proteins were analysed via western blot analysis and Ponceau staining, respectively. (d) The lysates prepared from H1299 cells after treatment with 25 μM MG132 for 8 h were subject to immunoprecipitation with anti-ARF antibody. The immunoprecipitates were analysed via western blot analysis with anti-Siva1 antibody. (e) The subcellular localization of endogenously expressed ARF and Siva1. H1299 cells were immunostained with anti-ARF and anti-Siva1 antibodies followed by rhodamine-conjugated anti-rabbit and fluorescein isothiocyanate (FITC)-conjugated anti-mouse IgG. The nucleus was also visualized using Hoechst 33342 staining. (f) Subcellular localization of exogenous Flag-Siva1 and endogenous ARF. H1299 cells seeded on coverslides were transfected with or without Flag-Siva1. Twenty-four hours after transfection, cells were treated with or without MG132 for another 6 h as indicated, fixed with 4% paraformaldehyde in PBS. The cells were then immunostained with anti-Flag and anti-ARF antibodies followed by rhodamin-conjugated anti-mouse and FITC-conjugated anti-rabbit IgG. The images were acquired using a confocal microscope. (g) The subcellular localization of exogenous Flag-Siva1 and GFP-ARF in HeLa cells. HeLa cells expressing GFP, GFP-ARF and Flag-Siva1 either individually or in combination were immunostained with anti-Flag antibody followed by rhodamine-conjugated anti-mouse IgG. The nucleus was also stained with Hoechst 33342. The images were acquired using a confocal microscope. The cellular distribution of ARF protein in the presence or absence of Siva1 was also analysed using NIS-Elements BR3.1 software (Nikon, Japan) based on the fluorescence intensity. The data are shown as the mean±s.d. based on ~50 analyzed nuclei. Figure 1: Siva1 is a novel ARF-binding partner. ( a ) H1299 cells were co-transfected with Flag-Siva1 and GFP-ARF as indicated. Twenty-four hours after transfection, cells were treated with 25 μM MG132 for an additional 8 h. The cell lysates were immunoprecipitated with anti-Flag antibody followed by western blot analysis with the indicated antibodies. HC and LC indicate the IgG heavy chain and the IgG light chain, respectively. ( b ) H1299 cells were co-transfected with GFP-Siva1 and Flag-ARF. Twenty-four hours post transfection, the cells were treated with 25 μM MG132 for an additional 8 h. The cell lysates were subject to immunoprecipitation with anti-Flag antibody. The immunoprecipitates were analysed via western blot analysis. HC indicates the IgG heavy chain. ( c ) The purified GST and GST-ARF proteins were incubated separately with recombinant Flag-Siva1 protein purified from HEK293T cells. Bead-bound and input proteins were analysed via western blot analysis and Ponceau staining, respectively. ( d ) The lysates prepared from H1299 cells after treatment with 25 μM MG132 for 8 h were subject to immunoprecipitation with anti-ARF antibody. The immunoprecipitates were analysed via western blot analysis with anti-Siva1 antibody. ( e ) The subcellular localization of endogenously expressed ARF and Siva1. H1299 cells were immunostained with anti-ARF and anti-Siva1 antibodies followed by rhodamine-conjugated anti-rabbit and fluorescein isothiocyanate (FITC)-conjugated anti-mouse IgG. The nucleus was also visualized using Hoechst 33342 staining. ( f ) Subcellular localization of exogenous Flag-Siva1 and endogenous ARF. H1299 cells seeded on coverslides were transfected with or without Flag-Siva1. Twenty-four hours after transfection, cells were treated with or without MG132 for another 6 h as indicated, fixed with 4% paraformaldehyde in PBS. The cells were then immunostained with anti-Flag and anti-ARF antibodies followed by rhodamin-conjugated anti-mouse and FITC-conjugated anti-rabbit IgG. The images were acquired using a confocal microscope. ( g ) The subcellular localization of exogenous Flag-Siva1 and GFP-ARF in HeLa cells. HeLa cells expressing GFP, GFP-ARF and Flag-Siva1 either individually or in combination were immunostained with anti-Flag antibody followed by rhodamine-conjugated anti-mouse IgG. The nucleus was also stained with Hoechst 33342. The images were acquired using a confocal microscope. The cellular distribution of ARF protein in the presence or absence of Siva1 was also analysed using NIS-Elements BR3.1 software (Nikon, Japan) based on the fluorescence intensity. The data are shown as the mean±s.d. based on ~50 analyzed nuclei. Full size image To further confirm that Siva1 interacts with ARF physiologically, an endogenous co-immunoprecipitation assay was performed. As shown in Fig. 1d , Siva1 was readily detected in the immunoprecipitates with anti-ARF antibody but not with the control mouse IgG. The subsequent immunofluorescence analysis of endogenously expressed ARF and Siva1 showed that ARF was primarily localized in the nucleoli, while Siva1 was predominantly present in the nucleoplasm ( Fig. 1e ). However, in the presence of ectopically expressed Flag-Siva1, ARF was partially relocalized from the nucleoli to the nucleoplasm, as revealed by both immunofluorescence and western blot analyses ( Fig. 1f ; Supplementary Figs S1a,b ). These results suggest that Siva1 promotes the nucleoplasmic distribution of ARF, and taken together, these experimental results suggest that Siva1 physically interacts with ARF in the nucleoplasm. Structural determinants of the ARF-Siva1 interaction To identify the regions of Siva1 that are responsible for its interaction with ARF, we generated a panel of Siva1 deletion mutants ( Fig. 2a ). These mutants were individually co-transfected into HEK 293T cells together with Flag-ARF. A co-immunoprecipitation assay was then performed to evaluate the ARF-binding ability of these mutants. As shown in Fig. 2b , both Siva1ΔN and Siva1ΔDDHR displayed a strong interaction with ARF protein, while Siva1ΔC showed no interaction, thereby suggesting that the C-terminal domain of Siva1 is essential for its interaction with ARF. Similarly, we also generated a series of ARF deletion mutants and performed the co-immunoprecipitation assay to determine the regions of ARF that mediate binding with Siva1 ( Fig. 2c ). As shown in Fig. 2d , deletion of the C-terminal domain (ARFN64) did not affect the ARF-Siva1 interaction, while removal of the N-terminal 64 amino acids (ARFΔN64) almost completely abolished the ability of ARF to bind to Siva1. Additionally, removal of the N-terminal 20 amino acids (ARFΔN20) decreased the binding ability of ARF to Siva1. These data indicate that residues 1–20 of ARF are involved in the binding to Siva1, while residues 21–64 of ARF are required for its association with Siva1. Taken together, these results suggest that the ARF-Siva1 interaction involves the C terminus of Siva1 and the N terminus of ARF. 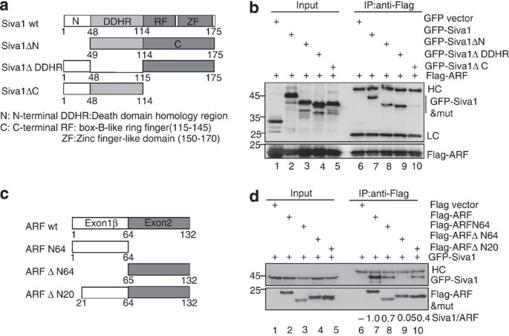Figure 2: Mapping of interaction regions between Siva1 and ARF. (a) A schematic representation of Siva1 and the corresponding mutants. (b) GFP-tagged wild-type Siva1 and the corresponding deletion mutants were individually transfected in HEK 293T cells with Flag-ARF. Twenty-four hours after transfection, the cells were treated with 25 μM MG132 for an additional 8 h. The cells lysates were then immunoprecipitated with anti-Flag antibody followed by western blot analysis. (c) Schematic representation of ARF and the corresponding mutants. (d) Flag-tagged wild-type ARF and the corresponding deletion mutants were individually transfected in HEK 293T cells with GFP-Siva1. Twenty-four hours after transfection, the cells were treated with 25 μM MG132 for an additional 8 h. The cell lysates were then subject to immunoprecipitation with anti-Flag antibody. The immunoprecipitates were analysed via western blot analysis. The protein bands were quantified using Gel-Pro analyser software. Of note, Flag-ARFΔN20 unexpectedly migrated faster than Flag-ARFΔN64 on the protein gel for unknown reasons. Figure 2: Mapping of interaction regions between Siva1 and ARF. ( a ) A schematic representation of Siva1 and the corresponding mutants. ( b ) GFP-tagged wild-type Siva1 and the corresponding deletion mutants were individually transfected in HEK 293T cells with Flag-ARF. Twenty-four hours after transfection, the cells were treated with 25 μM MG132 for an additional 8 h. The cells lysates were then immunoprecipitated with anti-Flag antibody followed by western blot analysis. ( c ) Schematic representation of ARF and the corresponding mutants. ( d ) Flag-tagged wild-type ARF and the corresponding deletion mutants were individually transfected in HEK 293T cells with GFP-Siva1. Twenty-four hours after transfection, the cells were treated with 25 μM MG132 for an additional 8 h. The cell lysates were then subject to immunoprecipitation with anti-Flag antibody. The immunoprecipitates were analysed via western blot analysis. The protein bands were quantified using Gel-Pro analyser software. Of note, Flag-ARFΔN20 unexpectedly migrated faster than Flag-ARFΔN64 on the protein gel for unknown reasons. Full size image Siva1 promotes ARF degradation Our immunofluorescence data showed that the ectopic expression of Siva1 leads to a dramatic decrease in endogenous ARF immunofluorescence intensity, which was significantly reversed by treatment with MG132 ( Fig. 1f ). This finding strongly indicates that Siva1 may promote the proteasome-dependent degradation of ARF. To test this idea, Flag-ARF was cointroduced into cells with increasing concentrations of expression plasmid encoding either GFP-Siva1 or GFP-Siva1ΔC. Western blot analysis showed that Siva1 abated ARF protein levels in a dose-dependent manner ( Fig. 3a , lanes 4–6). However, the ARF-binding-deficient mutant Siva1ΔC displayed no effect on ARF protein expression ( Fig. 3a , lanes 7–9). Additionally, with the increasing expression of Siva1 but not Siva1ΔC, the protein levels of endogenous ARF were concomitantly decreased ( Fig. 3b ). Additionally, when Siva1 expression was induced in H1299 cells via Nutlin-3 treatment, ARF protein levels were concurrently decreased ( Fig. 3c ). We next knocked down Siva1 in H1299 cells using small interference (si) RNA, which led to a significant increase in the levels of endogenous ARF ( Fig. 3d , lanes 1–3). The knockdown of ULF (a control), an E3 ligase of ARF, also led to an increase in ARF protein levels ( Fig. 3d , lane 1 versus 4). To further determine whether Siva1 decreases the half-life of ARF protein, GFP-ARF was coexpressed in H1299 cells either with or without Flag-Siva1. The ectopic expression of Siva1 noticeably shortened the half-life of ARF from ~4 to 2 h ( Fig. 3e ). In contrast, when Siva1 was knocked down, the half-life of ARF was dramatically prolonged from ~4 h to >9 h ( Fig. 3g ). Interestingly, this inhibitory effect of Siva1 on ARF stability was diminished when cells were treated with the proteasome inhibitor MG132 ( Fig. 3f ), thereby suggesting that Siva1 promotes ARF degradation via the proteasome pathway. 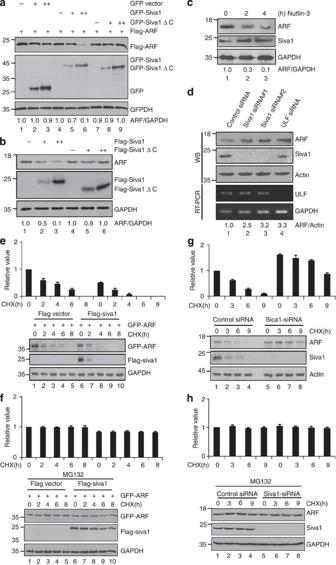Figure 3: Siva1 accelerates ARF degradation. (a) H1299 cells were co-transfected with Flag-ARF and increasing concentrations of either GFP-Siva1 or GFP-Siva1ΔC as indicated. The cell lysates were analysed via western blot analysis. Glyceraldehyde-3-phosphate dehydrogenase (GAPDH) was used as a loading control. The protein bands were quantified using Gel-Pro analyser software (USA). (b) H1299 cells were transfected with increasing concentrations of Flag-Siva1 or Flag-Siva1ΔC. The cell lysates were analysed via western blot analysis. Actin was used as a loading control. The protein bands were quantified using Gel-Pro analyser software. (c) H1299 cells were serum starved for 24 h. The cells were then treated with Nutlin-3 (60 μM) for the indicated periods of time and subsequently analysed via western blot analysis. The protein bands were quantified using Gel-Pro analyser software. (d) H1299 cells were transfected with control siRNA, Siva1-siRNA#1, Siva1-siRNA#2 or ULF-siRNA. Forty-eight hours after transfection, the cell lysates were subject to western blot analysis with the indicated antibodies. The protein bands were quantified using Gel-Pro analyser software. Successful knockdown of ULF was confirmed via semi-quantitative RT-PCR (PCR with reverse transcription) analysis. (e,f) H1299 cells were co-transfected with GFP-ARF plus either Flag-Siva1 or control vector. Twenty-four hours after transfection, the cells were treated either without (e) or with (f) MG132 (25 μM) for an additional 4 h, and CHX (20 μg ml−1) was then added to the medium for the indicated periods of time. Protein expression was analysed via western blot analysis. The normalized quantity of GFP-ARF is also shown. The data are represented as the mean±s.d. of three independent experiments. (g,h) H1299 cells were transfected with control siRNA or Siva1-siRNA. Forty-eight hours later, the cells were treated either without (g) or with (h) MG132 (25 μM) for 4 h and CHX (20 μg ml−1) for the indicated periods of time. The expression levels of ARF and Siva1 were determined via western blot analysis. The normalized quantity of ARF is also shown. The data are represented as the mean±s.d. of three independent experiments. Figure 3: Siva1 accelerates ARF degradation. ( a ) H1299 cells were co-transfected with Flag-ARF and increasing concentrations of either GFP-Siva1 or GFP-Siva1ΔC as indicated. The cell lysates were analysed via western blot analysis. Glyceraldehyde-3-phosphate dehydrogenase (GAPDH) was used as a loading control. The protein bands were quantified using Gel-Pro analyser software (USA). ( b ) H1299 cells were transfected with increasing concentrations of Flag-Siva1 or Flag-Siva1ΔC. The cell lysates were analysed via western blot analysis. Actin was used as a loading control. The protein bands were quantified using Gel-Pro analyser software. ( c ) H1299 cells were serum starved for 24 h. The cells were then treated with Nutlin-3 (60 μM) for the indicated periods of time and subsequently analysed via western blot analysis. The protein bands were quantified using Gel-Pro analyser software. ( d ) H1299 cells were transfected with control siRNA, Siva1-siRNA#1, Siva1-siRNA#2 or ULF-siRNA. Forty-eight hours after transfection, the cell lysates were subject to western blot analysis with the indicated antibodies. The protein bands were quantified using Gel-Pro analyser software. Successful knockdown of ULF was confirmed via semi-quantitative RT-PCR (PCR with reverse transcription) analysis. ( e , f ) H1299 cells were co-transfected with GFP-ARF plus either Flag-Siva1 or control vector. Twenty-four hours after transfection, the cells were treated either without ( e ) or with ( f ) MG132 (25 μM) for an additional 4 h, and CHX (20 μg ml −1 ) was then added to the medium for the indicated periods of time. Protein expression was analysed via western blot analysis. The normalized quantity of GFP-ARF is also shown. The data are represented as the mean±s.d. of three independent experiments. ( g , h ) H1299 cells were transfected with control siRNA or Siva1-siRNA. Forty-eight hours later, the cells were treated either without ( g ) or with ( h ) MG132 (25 μM) for 4 h and CHX (20 μg ml −1 ) for the indicated periods of time. The expression levels of ARF and Siva1 were determined via western blot analysis. The normalized quantity of ARF is also shown. The data are represented as the mean±s.d. of three independent experiments. Full size image Siva1 is a novel E3 ubiquitin ligase of ARF To further investigate whether ubiquitin is involved in ARF degradation induced by Siva1, an in vivo ubiquitination assay was performed. As shown in Fig. 4a , the ectopic expression of Siva1 dramatically increased the polyubiquitination of both exogenous and endogenous ARF. In contrast, knockdown of Siva1 led to a decrease in the polyubiquitination of endogenous ARF ( Fig. 4c ). Polyubiquitination usually occurs at Lys 48 and Lys 63 of ubiquitin. It has been well recognized that Lys 48 -linked but not Lys 63 -linked polyubiquitination is involved in proteolysis. To examine whether Siva1 promotes Lys 48 -linked polyubiquitin chain formation of ARF, we performed an ubiquitination assay with an ubiquitin mutant, UbK48R, which cannot form Lys 48 -conjugated polyubiquitin chains. As shown in Fig. 4d , Siva1 strongly induced the polyubiquitination of ARF in the presence of wild-type ubiquitin but not K48R ubiquitin. As Siva1 contains a box-B-like ring finger domain and a zinc finger-like domain ( Fig. 2a ), we sought to determine whether Siva1 is an E3 ligase of ARF. To test this possibility, an in vitro ubiquitination assay was performed with purified recombinant proteins. As shown in Fig. 4f and Supplementary Fig. S2a , Siva1 promoted the polyubiquitination of ARF in a dose-dependent manner. However, compared with wild-type Siva1, the ARF-binding defective mutant, Siva1ΔC, failed to show any effect on the polyubiquitination of ARF ( Fig. 4g ). Collectively, these results suggest that Siva1 is a novel E3 ligase of ARF and induces the polyubiquitination and degradation of ARF. 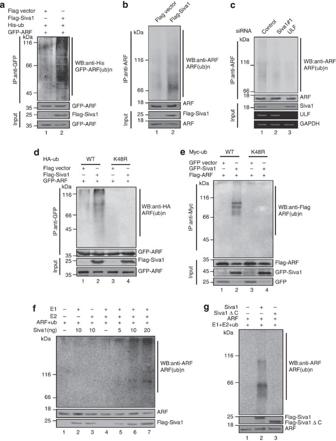Figure 4: Siva1 promotes the polyubiquitination of ARF. (a) H1299 cells were co-transfected with His-Ub, GFP-ARF and either Flag-Siva1 or control vector as indicated. Twenty-four hours after transfection, the cells were treated with MG132 (25 μM) for an additional 8 h. The cell lysates were immunoprecipitated with anti-GFP antibody followed by western blot analysis with the indicated antibodies. (b) H1299 cells were transfected either with or without Flag-Siva1. Twenty-four hours after transfection, the cells were treated with MG132 (25 μM) for an additional 8 h. The cell lysates were then immunoprecipitated with anti-ARF antibody followed by western blot analysis. (c) H1299 cells were transfected with control siRNA, Siva1-siRNA#1 or ULF-siRNA. Forty-eight hours later, the cells were treated with MG132 (25 μM) for an additional 8 h. The cell lysates were immunoprecipitated with anti-ARF antibody followed by western blot analysis. (d) H1299 cells were transfected with GFP-ARF, HA-UbWT, HA-UbK48R and Flag-Siva1 in the indicated combinations. The cells were then treated with MG132 (25 μM) for 8 h. The cell lysates were subject to immunoprecipitation followed by western blot analysis. (e) H1299 cells were transfected with Flag-ARF, pCW7 (Myc-UbWT), pCW8 (Myc-UbK48R) and GFP-Siva1 in the indicated combinations. Twenty-four hours after transfection, the cells were treated with MG132 (25 μM) for an additional 8 h. The cell lysates were then subject to immunoprecipitation followed by western blot analysis with the indicated antibodies. (f) ARF is ubiquitinated by Siva1in vitro.Purified Flag-ARF was mixed with E1 (10 ng), E2 (His-UbcH5a, 100 ng), Flag-ubiquitin (5 μg, Sigma), and increasing amounts of purified Flag-Siva1 in 10 μl of reaction buffer as indicated. The mixture was incubated at 37 °C for 3.5 h and then analysed via western blot analysis. (g) Purified Flag-ARF was mixed with E1 (10 ng), E2 (His-UbcH5a, 100 ng), Flag-ubiquitin (5 μg, Sigma), and either Flag-Siva1 or Flag-Siva1ΔC in 10 μl of reaction buffer. The mixture was incubated at 37 °C for 3.5 h and then analysed via western blot analysis with the indicated antibodies. Figure 4: Siva1 promotes the polyubiquitination of ARF. ( a ) H1299 cells were co-transfected with His-Ub, GFP-ARF and either Flag-Siva1 or control vector as indicated. Twenty-four hours after transfection, the cells were treated with MG132 (25 μM) for an additional 8 h. The cell lysates were immunoprecipitated with anti-GFP antibody followed by western blot analysis with the indicated antibodies. ( b ) H1299 cells were transfected either with or without Flag-Siva1. Twenty-four hours after transfection, the cells were treated with MG132 (25 μM) for an additional 8 h. The cell lysates were then immunoprecipitated with anti-ARF antibody followed by western blot analysis. ( c ) H1299 cells were transfected with control siRNA, Siva1-siRNA#1 or ULF-siRNA. Forty-eight hours later, the cells were treated with MG132 (25 μM) for an additional 8 h. The cell lysates were immunoprecipitated with anti-ARF antibody followed by western blot analysis. ( d ) H1299 cells were transfected with GFP-ARF, HA-UbWT, HA-UbK48R and Flag-Siva1 in the indicated combinations. The cells were then treated with MG132 (25 μM) for 8 h. The cell lysates were subject to immunoprecipitation followed by western blot analysis. ( e ) H1299 cells were transfected with Flag-ARF, pCW7 (Myc-UbWT), pCW8 (Myc-UbK48R) and GFP-Siva1 in the indicated combinations. Twenty-four hours after transfection, the cells were treated with MG132 (25 μM) for an additional 8 h. The cell lysates were then subject to immunoprecipitation followed by western blot analysis with the indicated antibodies. ( f ) ARF is ubiquitinated by Siva1 in vitro. Purified Flag-ARF was mixed with E1 (10 ng), E2 (His-UbcH5a, 100 ng), Flag-ubiquitin (5 μg, Sigma), and increasing amounts of purified Flag-Siva1 in 10 μl of reaction buffer as indicated. The mixture was incubated at 37 °C for 3.5 h and then analysed via western blot analysis. ( g ) Purified Flag-ARF was mixed with E1 (10 ng), E2 (His-UbcH5a, 100 ng), Flag-ubiquitin (5 μg, Sigma), and either Flag-Siva1 or Flag-Siva1ΔC in 10 μl of reaction buffer. The mixture was incubated at 37 °C for 3.5 h and then analysed via western blot analysis with the indicated antibodies. Full size image Siva1 negatively regulates the ARF-p53 pathway As Siva1 interacts with the N-terminal domain of ARF ( Fig. 2d ) and this domain is required for Mdm2 binding [4] , we sought to determine whether Siva1 interferes with the ARF-Mdm2 interaction. As shown in Supplementary Fig. S2b , the ectopic expression of wild-type Siva1 but not the ARF-binding defective mutant, Siva1ΔC, markedly decreased the interaction between ARF and Mdm2. Moreover, Siva1 inhibited the interaction between ARF and Mdm2 in a dose-dependent manner ( Supplementary Fig. S2c ). These results, together with the finding that Siva1 promotes ARF degradation, suggest that Siva1 may relieve the inhibitory effect of ARF on Mdm2 E3 ligase activity towards p53. To test this possibility, a co-transfection assay was performed in mouse embryonic fibroblast (MEF) cells deficient in both p53 and Mdm2. When Siva1 was coexpressed with ARF and p53 in these cells, it did not significantly alter the expression levels of p53 ( Fig. 5a , lanes 1–3). However, with the additional expression of Mdm2, Siva1 reduced the enhancing effect of ARF on p53 protein expression ( Fig. 5a , lane 5 versus 6). These data indicate that Siva1 regulates p53 expression in an Mdm2-dependent manner. As ARF and p53 are frequently mutated in cancer cells, generally in a mutually exclusive manner [20] , we next used a primary human fetal lung fibroblast cell line to further confirm the effect of Siva1 on the ARF-p53 pathway. As shown in Fig. 5b , knockdown of Siva1 resulted in a marked increase in p53 protein levels, which correlated well with the increased levels of ARF ( Fig. 5b lane 1 versus 2 and 5c lane 1 versus 2). However, the additional knockdown of ARF almost completely attenuated the inhibitory effect of Siva1 on p53 expression ( Fig. 5c , lane 3 versus 4), thereby suggesting that Siva1 negatively regulates p53 expression via ARF. Of note, Siva1 and ULF exhibited similar effects on p53 and ARF protein levels ( Fig. 5b , lanes 1–3). Together, these results indicate the important function of Siva1 in the regulation of the ARF–p53 axis. 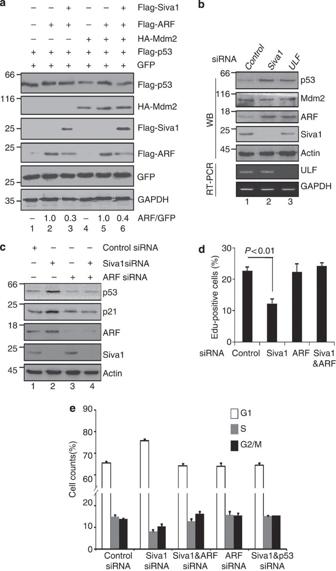Figure 5: Siva1 regulates the ARF–p53 axis. (a) Mdm2−/−p53−/−MEF cells were transfected with Flag-Siva1, Flag-ARF, Flag-Mdm2 and Flag-p53 in the indicated combinations. The cell lysates were subject to western blot analysis with the indicated antibodies. The protein bands were quantified using Gel-Pro analyser software. (b) Human fetal lung fibroblast cells were transfected with the indicated siRNAs. Forty-eight hours later, the cell lysates were analysed via western blot analysis. The knockdown efficiency of Siva1 and ULF was determined via western blot analysis and semi-quantitative RT–PCR analysis, respectively. (c) Human fetal lung fibroblast cells were transfected with the indicated siRNAs. Forty-eight hours later, the cell lysates were subject to western blot analysis. (d) Human fetal lung fibroblast cells were transfected with the indicated siRNAs. Forty-eight hours after transfection, the cells were stained with 5-ethynyl-2′-deoxyuridine (EdU). The percentage of EdU-positive cells were calculated, and the data are represented as the mean±s.d. of three independent experiments. (e) Human fetal lung fibroblast cells were transfected with the indicated siRNAs. Forty-eight hours later, the cells were harvested and analysed via flow cytometry. The data are shown as the mean±s.d. of three independent experiments. Figure 5: Siva1 regulates the ARF–p53 axis. ( a ) Mdm2 −/− p53 −/− MEF cells were transfected with Flag-Siva1, Flag-ARF, Flag-Mdm2 and Flag-p53 in the indicated combinations. The cell lysates were subject to western blot analysis with the indicated antibodies. The protein bands were quantified using Gel-Pro analyser software. ( b ) Human fetal lung fibroblast cells were transfected with the indicated siRNAs. Forty-eight hours later, the cell lysates were analysed via western blot analysis. The knockdown efficiency of Siva1 and ULF was determined via western blot analysis and semi-quantitative RT–PCR analysis, respectively. ( c ) Human fetal lung fibroblast cells were transfected with the indicated siRNAs. Forty-eight hours later, the cell lysates were subject to western blot analysis. ( d ) Human fetal lung fibroblast cells were transfected with the indicated siRNAs. Forty-eight hours after transfection, the cells were stained with 5-ethynyl-2′-deoxyuridine (EdU). The percentage of EdU-positive cells were calculated, and the data are represented as the mean±s.d. of three independent experiments. ( e ) Human fetal lung fibroblast cells were transfected with the indicated siRNAs. Forty-eight hours later, the cells were harvested and analysed via flow cytometry. The data are shown as the mean±s.d. of three independent experiments. Full size image To investigate the functional consequence of Siva1-mediated ARF and p53 regulation, we evaluated the effect of Siva1 on cell proliferation and cell cycle progression. As shown in Fig. 5d , knockdown of Siva1 effectively inhibited the proliferation of human fetal lung fibroblast cells, as revealed by a dramatic decrease in the number of 5-ethynyl-2′-deoxyuridine-positive cells (from 22.7 to 12.2%) via Siva1 knockdown. The additional knockdown of ARF completely reversed the decrease in proliferation of Siva1 knockdown cells ( Fig. 5d ). The subsequent flow cytometric analysis revealed that Siva1 knockdown induced cell cycle arrest by increasing the proportion of cells in the G1 phase (65 versus 76%), which was largely inhibited by concomitant knockdown of either ARF or p53 ( Fig. 5e ). Taken together, these results suggest that Siva1 is an important regulator of the ARF-p53 pathway. ARF, the second most frequently mutated tumour suppressor in human cancer, exerts multiple tumour suppressor functions, some of which are mediated by the p53 signalling pathway [21] . In this context, ARF is activated by various oncogenic insults [22] , [23] . Once activated, ARF binds to and inactivates Mdm2, which leads to the stabilization of p53 and subsequent tumour suppression. Additionally, emerging evidence suggests that ARF also displays p53-independent functions. The activation of ARF in p53-null cancer cells both leads to a significant inhibition of cell growth and promotes apoptosis [24] , [25] , [26] , [27] , [28] . Given the potent tumour-suppressive activity of ARF, cellular levels of ARF are strictly controlled by several mechanisms. For example, ARF is transcriptionally regulated by multiple factors [29] , [30] , [31] , [32] . Moreover, ARF is subject to ULF-mediated lysine-independent ubiquitination and subsequent rapid degradation [13] . However, the exact mechanism of ARF regulation remains largely unknown. In this study, we describe Siva1 as a novel E3 ligase of ARF. Siva1 physiologically interacts with ARF both in vitro and in vivo . Additionally, the ectopic expression of Siva1 reduces ARF stability, while knockdown of Siva1 increases ARF stability. More importantly, Siva1 regulates cell cycle progression and cell proliferation in an ARF/p53-dependent manner. These results suggest that Siva1 plays an important role in the control of ARF stability, thereby repressing ARF and p53 function in unstressed cells. Given the low expression of ARF under physiological conditions and the induced expression of ARF upon oncogenic stress, it would be interesting to determine whether oncogenic signals disrupt the Siva1–ARF interaction and thus lead to the upregulation of ARF. If this is the case, what are these signals? The dysregulation of ARF has been implicated in various human diseases, such as cancer, aging and diabetics [9] , [33] , [34] . Another interesting issue concerns whether Siva1 is also involved in these diseases, acting by repressing ARF expression. A recent study has suggested that ARF is fairly stable in the nucleolus but turns over rapidly in the nucleoplasm [11] . Consistent with this finding, our immunofluorescence and western blot analysis results show that ectopically expressed Siva1 promotes ARF nucleoplasmic distribution where ARF is ubiquitinated and degraded by Siva1; however, whether this occurs under physiological conditions remains to be further characterized. Moreover, Siva1 specifically promotes the Lys 48 -linked polyubiquitin chain formation of ARF. As the human ARF protein has no lysines, ubiquitin modification of ARF promoted by Siva1 may occur via a lysine-independent mechanism. Deletion analyses reveal that the C terminus of Siva1 is essential for binding to ARF. The direct binding of Siva1 to ARF appears to be required for the rapid degradation of ARF, as supported by the finding that the mutant Siva1ΔC, which is unable to interact with ARF, has no effect on the stability and ubiquitination of ARF. Additionally, we show that the N-terminal domain (amino acids 1–20) of ARF is involved in its interaction with Siva1, but is not essential for this association. As this N terminus (amino acids 2–14) has been well recognized as a critical region for binding to Mdm2, it is not surprising to see that Siva1 could compete with Mdm2 to bind to ARF. By this way, Siva1 may relieve the inhibitory effect of ARF on Mdm2, thereby facilitating Mdm2-mediated p53 degradation. Of note, there may be only a partial competition between Siva1 and Mdm2 for ARF binding ( Supplementary Fig. S2b ) as Siva1 binds to residues 21–64 in addition to residues 1–20 of ARF. Importantly, residue 21–64 of ARF is found to be essential for Siva1 binding, and through this binding, Siva1 directly promotes ARF ubiquitination and degradation. Thus, Siva1 may negatively regulate p53 expression through at least two mechanisms: the impeded interaction between ARF and Mdm2 and the accelerated degradation of ARF. Our recent study has suggested that Siva1 enhances Mdm2-mediated p53 degradation and suppresses p53-mediated gene expression and apoptosis [18] . In this report, we also provide strong evidence that Siva1 regulates the Mdm2-p53 pathway by targeting ARF for degradation. These findings indicate that Siva1 is a negative regulator of the Mdm2-p53 pathway. Therefore, it is not surprising that the downregulation of Siva1 greatly inhibits tumour formation in xenograft models [18] . Intriguingly, we have recently shown that the upregulation of Siva1 suppresses both the epithelial–mesenchymal transition (EMT) and the metastasis of tumour cells by regulating stathmin function, while knockdown of Siva1 enhances these effects [35] . This finding suggests that Siva1 functions as a suppressor of tumour metastasis. Consistent with this notion, metastatic breast tumours indeed express lower levels of Siva1 than low metastatic breast tumors [35] . Taken together, it appears that Siva1 might be a two-faced player functioning in different stages of tumorigenesis; further detailed analysis is needed before the role of Siva1 in the regulation of tumorigenesis can be fully characterized. Reagents The following antibodies were used in this study: GFP (Sigma, MO), Flag (Sigma, MO), GAPDH (Cell Signaling, MA), Myc (Abmart), Siva1 (Abnova), ARF (NeoMarkers), Fibrillarin (Abgent), Lamin B1 (Santa Cruz Biotechnology), Mdm2 (Santa Cruz Biotechnology), p53 (Calbiochem and Santa Cruz Biotechnology) and NPM/B23 (Sigma). Hoechst 33342, MG132, CHX, Nutlin-3, anti-Flag M2 affinity gel and 3 × Flag peptide were purchased from Sigma. Cell culture and transfection H1299, HEK293T, HeLa, wild-type MEF and p53 −/− Mdm2 −/− MEF cells were maintained in Dulbecco’s modified Eagle’s medium (Invitrogen, CA) with 10% fetal bovine serum. Human fetal lung fibroblast cells were purchased from CHI SCIENTIFIC (Jiangsu, China) and maintained in Dulbecco’s modified Eagle’s medium with fetal bovine serum, HEPES, penicillin and streptomycin. The transfection assay using Lipofectamin 2000 (Invitrogen, CA) was performed according to the instructions recommended by the manufacturer. siRNA-mediated knockdown The transfection of siRNA was performed as previously described [36] . The following siRNA duplexes were obtained from GenePharma (Shanghai, China): Siva1-siRNA#1 (5′-UUUCUCGUACAUGUCACUG-3′), ULF-siRNA (5′-GGUAGUGACUCCACCCAUUUU-3′, 5′-GAACACAGAUGGUGCGAUAUU-3′, and 5′-GAACACAGAUGGUGCGAUAUU-3′), p14 ARF -siRNA (5′-GAUCAUCAGUCACCGAAGGUU-3′), and control siRNA (5′-GACAAAGACUCAUACAAUAUU-3′). Siva1-siRNA#2 and p53-siRNA were purchased from Santa Cruz Biotechnology (USA). Co-immunoprecipitation Cells were treated with MG132 for 6–8 h and then lysed with immunoprecipitation (IP) lysis buffer (50 mM Tris–HCl PH 8.0, 150 mM NaCl, 1% NP40 and 0.5% deoxycholate acid) supplemented with 1 × cocktail. The cell lysates were incubated with antibody-conjugated protein A/G beads overnight at 4 °C. The immunoprecipitates were washed with ice-cold PBS and boiled in sample buffer at 100 °C. The samples were resolved via SDS–polyacrylamide gel electrophoresis and probed using the indicated antibodies. Western blot and immunofluorescence analyses Western blot and immunofluorescence analyses were performed as described previously [18] . Protein purification To purify the recombinant ARF and Siva1 proteins, Flag-ARF or Flag-Siva1 was transfected into HEK293T cells. Next, 24 h after transfection, the cell lysates were immunoprecipitated with anti-Flag M2 affinity beads (Sigma). The beads were washed extensively via sequential washes with IP lysis buffer containing 0.25, 0.5 and 1 M KCl to remove the non-specific binding proteins. Proteins were then eluted from the beads with 3 × Flag peptide (Sigma). The eluted protein concentration was determined using a BCA kit. In vivo ubiquitination Cells were treated with MG132 for 8 h before collection and then lysed in SDS lysis buffer (50 mM Tris pH 6.8, 1% SDS, 10% glycerol, 150 mM NaCl and protease inhibitors). After boiling for 5 min, whole cell lysates were diluted 10 times with cold IP lysis buffer and subject to immunoprecipitation with the indicated antibodies. The immunoprecipitates were analysed via western blot analysis to assess ARF polyubiquitination. In vitro ubiquitination The in vitro ubiquitination assay was performed as described previously [13] , [37] . Briefly, the purified recombinant proteins Flag-ARF and Flag-Siva1 were mixed with the other components, including E1 (Sigma, 10 ng), E2 (His-UbcH5a, Boston Biochem, 100 ng) and Flag-ubiquitin (Sigma, 5 μg) in 10 μl of reaction buffer (40 mM Tris–HCl pH 7.6, 5 mM MgCl 2 , 2 mM ATP, and 2 mM DTT). The mixture was incubated at 37 °C for 3.5 h and then analysed via western blotting. Nucleoli purification The purification of nucleoli was performed as described previously [38] . Flow cytometric analysis Cell cycle distribution was analysed using a FACScalibur flow cytometer (BD Biosciences, CA). Briefly, cells were seeded in six-well plates at 30–50% confluency and transfected with the indicated siRNAs. Next, 24 h after transfection, the cells were collected, stained with PI solution, and analysed via flow cytometry. Data analysis was performed using WinMDI 2.9 software (The Scripps Research Institute, CA). How to cite this article: Wang, X. et al . Siva1 inhibits p53 function by acting as an ARF E3 ubiquitin ligase. Nat. Commun. 4:1551 doi: 10.1038/ncomms2533 (2013).